Direct observation of lattice symmetry breaking at the hidden-order transition in URu2Si2 Since the 1985 discovery of the phase transition at T HO =17.5 K in the heavy-fermion metal URu 2 Si 2 , neither symmetry change in the crystal structure nor large magnetic moment that can account for the entropy change has been observed, which makes this hidden order enigmatic. Recent high-field experiments have suggested electronic nematicity that breaks fourfold rotational symmetry, but direct evidence has been lacking for its ground state in the absence of magnetic field. Here we report on the observation of lattice symmetry breaking from the fourfold tetragonal to twofold orthorhombic structure by high-resolution synchrotron X-ray diffraction measurements at zero field, which pins down the space symmetry of the order. Small orthorhombic symmetry-breaking distortion sets in at T HO with a jump, uncovering the weakly first-order nature of the hidden-order transition. This distortion is observed only in ultrapure samples, implying a highly unusual coupling nature between the electronic nematicity and underlying lattice. Interacting electrons in solids can generate a rich variety of phase transitions. The most essential step for elucidating the nature of a phase transition is to identify which symmetries are broken in the ordered phase. In the heavy-fermion metal URu 2 Si 2 (refs 1 , 2 , 3 ), tremendous efforts have been made to understand the properties of the hidden-order phase transition at T HO =17.5 K, but its nature has been a long-standing mystery [4] . Recently, magnetic torque [5] , cyclotron resonance [6] , [7] and nuclear magnetic resonance (NMR) [8] measurements have suggested the occurrence of rotational symmetry breaking below T HO , which points to an electronic nematic order with in-plane anisotropy elongated along the [110] direction. These measurements, however, have been carried out under in-plane magnetic fields and hence we cannot rule out the possibility that the observed symmetry breaking is induced by the applied magnetic field. Direct determination of the crystal symmetry in the absence of field is therefore absolutely requisite to obtain the conclusive evidence of the rotational symmetry breaking in the hidden-order phase. Owing to the electromagnetic interaction of conduction electrons with ions of the lattice, when the electrons in a metal undergo the transition to a state that breaks one of the space symmetries of the crystal, the same symmetry breaking of the underlying lattice is expected to occur. Generally, the symmetry of the low-temperature ordered phase should be lower than but belong to a subgroup of the symmetry above the transition temperature. In the high-temperature disordered phase, URu 2 Si 2 has a body-centred tetragonal crystal structure ( Fig. 1a,d ) belonging to the I 4/ mmm symmetry group (No. 139 in the international tables for crystallography), which has 15 maximal non-isomorphic subgroups. Recent quantum oscillations [9] and angle-resolved photoemission spectroscopy [10] , [11] , [12] studies have revealed that the electronic structure in the hidden-order phase is similar to that of antiferromagneitc phase under pressure. This implies that in the hidden-order phase the Brillouin Zone is folded with the antiferroic wave vector Q =(001) and the nested parts of Fermi surface are gapped as in the antiferromagnetic phase [13] . In such a case, the magnetic space (two-colour crystallographic) group is lowered from the body-centred to a simple tetragonal type. However, the crystal structure symmetry ignoring the local electronic distributions (that is, spin or orbital directions) does not change, and thus the space group that can be determined by X-ray Bragg diffraction remains to be I 4/ mmm . 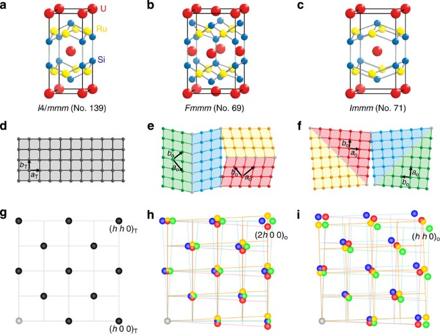Figure 1: Crystals structure of URu2Si2above and below the hidden-order transition. (a) Body-centred tetragonalI4/mmmstructure aboveTHO. (b) OrthorhombicFmmmstructure revealed by the present study in the hidden-order phase belowTHO. (c) Another orthorhombicImmmstructure with broken fourfold symmetry, which belongs to a subgroup ofI4/mmm, is shown for a comparison. Thin solid line indicates the unit cell. (d–f), Schematic U atom arrangements in the basal plane for each structure, and formation of four degenerate domains sketched by different colours. In-plane primitive vectors are indicated by arrows. (g–i) Bragg points in thel=0 plane forh,k⩾0. The domain formation splits the Bragg points into three or four points, depending on the Miller index20,21. Figure 1: Crystals structure of URu 2 Si 2 above and below the hidden-order transition. ( a ) Body-centred tetragonal I 4/ mmm structure above T HO . ( b ) Orthorhombic Fmmm structure revealed by the present study in the hidden-order phase below T HO . ( c ) Another orthorhombic Immm structure with broken fourfold symmetry, which belongs to a subgroup of I 4/ mmm , is shown for a comparison. Thin solid line indicates the unit cell. ( d – f ), Schematic U atom arrangements in the basal plane for each structure, and formation of four degenerate domains sketched by different colours. In-plane primitive vectors are indicated by arrows. ( g – i ) Bragg points in the l =0 plane for h , k ⩾ 0. The domain formation splits the Bragg points into three or four points, depending on the Miller index [20] , [21] . Full size image If the fourfold rotational symmetry is broken in the hidden-order phase, the crystal structure itself is expected to have an orthorhombic distortion, lowering the space symmetry. For I 4/ mmm , two subgroups Fmmm (No. 69, Fig. 1b,e ) and Immm (No. 71, Fig. 1c,f ) may have such orthorhombic distortions, but the ab plane primitive vector direction is rotated 45° with respect to each other. These motivate us to study ( hh 0) T Bragg diffraction peaks at zero field that are most sensitive to the Fmmm -type orthorhombicity ( Fig. 1g–i ), which is compatible with the putative in-plane anisotropy elongated along the [110] directions. Based on the synchrotron measurements in a ultraclean sample using optimized conditions that have not been tried before, here we report on the observation of the orthorhombic distortion in the hidden-order phase of URu 2 Si 2 . Synchrotron X-ray diffraction We use two crystals with different purities evaluated by the residual resistivity ratio (RRR); one is a crystal with RRR~10, which is a typical value for crystals used in the previous studies [4] and the other is a new-generation ultraclean crystal with RRR~670 (refs 6 , 14 ). Here we checked crystalline quality by X-ray diffraction at room temperature and selected ones with the sharpest Bragg peaks ( Fig. 2a ), which ensures minimal strain effects inside the sample. Synchrotron X-ray diffraction at SPring-8 was used to analyse the crystal structure in the hidden-order phase of these crystals (see Methods). In order to achieve a very high resolution, we focus on a high-angle Bragg peak (880) T at which our experimental resolution of lattice spacing is as good as Δ d / d ~3 × 10 −5 ( Fig. 2b ). Moreover, to obtain bulk information, we tune the synchrotron X-ray energy at ~17.15 keV just below a uranium absorption edge, where X-ray attenuation length is more than 30 μm ( Fig. 2c ). 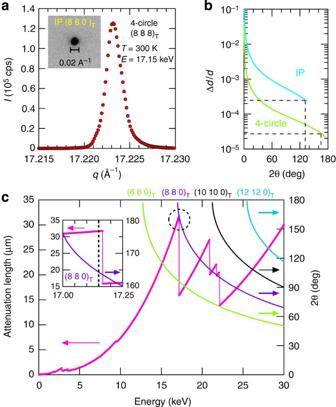Figure 2: High-resolution synchrotron X-ray diffraction measurements of URu2Si2single crystals. (a) (880) Bragg peak intensityI(q) of the ultrapure crystal measured with 17.15 keV X-ray (0.723 Å wave length) by a four-circle diffractometer at room temperature. Inset is an image of the (880) peak of the same sample taken by an IP with 18.8 keV X-ray. (b) Comparison between the estimated lattice spacing resolutions Δd/dfor the IP and the four-circle diffractometer (with angle resolutions Δ2θof 0.03° and 0.008°, respectively). Dashed lines mark the limits for available 2θangle spaces and the corresponding resolutions for each experimental apparatus. (c) Energy dependence of X-ray attenuation length and the scattering angle 2θ(right axis) for several (hh0) peaks of URu2Si2. Inset is an expanded view near the peak in the attenuation length around 17.15 keV marked by the dashed circle in the main panel. Figure 2: High-resolution synchrotron X-ray diffraction measurements of URu 2 Si 2 single crystals. ( a ) (880) Bragg peak intensity I ( q ) of the ultrapure crystal measured with 17.15 keV X-ray (0.723 Å wave length) by a four-circle diffractometer at room temperature. Inset is an image of the (880) peak of the same sample taken by an IP with 18.8 keV X-ray. ( b ) Comparison between the estimated lattice spacing resolutions Δ d / d for the IP and the four-circle diffractometer (with angle resolutions Δ2 θ of 0.03° and 0.008°, respectively). Dashed lines mark the limits for available 2 θ angle spaces and the corresponding resolutions for each experimental apparatus. ( c ) Energy dependence of X-ray attenuation length and the scattering angle 2 θ (right axis) for several ( hh 0) peaks of URu 2 Si 2 . Inset is an expanded view near the peak in the attenuation length around 17.15 keV marked by the dashed circle in the main panel. Full size image One-dimensional diffraction profiles In Fig. 3a , we show the temperature dependence of the (880) T Bragg intensity as a function of the magnitude of the scattering vector q , which is measured by the 2 θ / θ mode corresponding to scans along the radial direction from the origin in the reciprocal space. At high temperatures above T HO , in both crystals we have a single peak with a narrow width. From the full width at half maximum, the distribution of lattice constant is estimated as δa / a ~1.3(3) × 10 −4 , which is more than a factor of 3 smaller than that in the previous studies [15] , [16] , [17] , indicating very high crystalline quality of our samples. Upon entering the hidden-order phase below T HO , the data for RRR~10 sample shows no significant change in its shape, but for much cleaner sample with RRR~670 the single peak above T HO suddenly changes to a broadened shape with clear splitting. At low temperatures the split peaks can be reasonably fitted to two Gaussian peaks ( Fig. 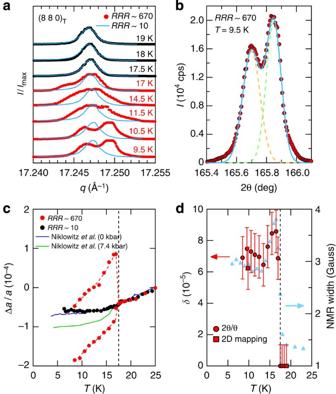Figure 3: Temperature dependence of the (880)TBragg peak in URu2Si2. (a) IntensityInormalized by the peak valueImaxas a function of scattering vectorqfor two samples with different RRR values (blue lines for RRR~10, black (T>THO) and red (T<THO) circles for RRR~670). Each curve is shifted vertically for clarity. (b) The data at 9.5 K belowTHO(circles) can be fitted to a sum (solid line) of two Gaussian functions with different lattice constantsaO≈5.8290 Å andbO≈5.8281 Å (dashed lines). (c) Temperature dependence of lattice constants Δa(T)=a(T)−a(25 K) (circles) compared with the previous report at ambient pressure (hidden-order phase) and at high pressure (antiferromagnetic phase)15. Dashed lines are guides for the eyes. (d) The orthorhombicityδ=(aO−bO)/(aO+bO) estimated from the two-peak fitting as a function of temperature (red circles). The orthorhombicity estimated from the 2D mapping at 10 K (Fig. 4) is also plotted (red squares). Error bars represents the X-ray experimental resolution. The temperature dependence of the NMR line width for in-plane field (S. Kambe, personal communication) is plotted for comparison (blue triangles, right axis). The dashed line marks the transition temperatureTHO=17.5 K. 3b ) with the widths comparable to the high-temperature data above T HO , from which the orthorhombicity Figure 3: Temperature dependence of the (880) T Bragg peak in URu 2 Si 2 . ( a ) Intensity I normalized by the peak value I max as a function of scattering vector q for two samples with different RRR values (blue lines for RRR~10, black ( T > T HO ) and red ( T < T HO ) circles for RRR~670). Each curve is shifted vertically for clarity. ( b ) The data at 9.5 K below T HO (circles) can be fitted to a sum (solid line) of two Gaussian functions with different lattice constants a O ≈5.8290 Å and b O ≈5.8281 Å (dashed lines). ( c ) Temperature dependence of lattice constants Δ a ( T )= a ( T )− a (25 K) (circles) compared with the previous report at ambient pressure (hidden-order phase) and at high pressure (antiferromagnetic phase) [15] . Dashed lines are guides for the eyes. ( d ) The orthorhombicity δ =( a O − b O )/( a O + b O ) estimated from the two-peak fitting as a function of temperature (red circles). The orthorhombicity estimated from the 2D mapping at 10 K ( Fig. 4 ) is also plotted (red squares). Error bars represents the X-ray experimental resolution. The temperature dependence of the NMR line width for in-plane field (S. Kambe, personal communication) is plotted for comparison (blue triangles, right axis). The dashed line marks the transition temperature T HO =17.5 K. Full size image is estimated, where a O and b O are the orthorhombic lattice constants, and 2 θ 1 and 2 θ 2 are the two-peak angles. The change in the lattice constant a for RRR~10 sample is consistent with the previous high-resolution Larmor diffraction measurements of (400) T Bragg peak for a similar RRR~10 sample [15] at ambient pressure ( Fig. 3c ). In sharp contrast, our new data on the ultraclean sample clearly shows a splitting into two different lattice constants a O and b O below T HO , evidencing the transition to the orthorhombic state. We note that these lattice constants do not track the data for the antiferromagnetic phase under pressure [15] and rather show an opposite trend that the averaged constant increases just below T HO . This indicates that our splitting cannot be explained by some inclusion of antiferromagnetic phase induced by local strain inside the sample, although there are different views on the origin of the small antiferromagnetic signals found in the neutron-scattering experiments [15] , [16] . In any case, the comparable intensities of the two peaks imply that the volumes of the corresponding parts are similar inside the crystal, which is not compatible with such an impurity-related origin of the peak splitting. We will discuss the implications of the crystal-purity dependence later, and now we focus on the data of the ultraclean sample. The temperature dependence of the orthorhombicity δ is demonstrated in Fig. 3d . The orthorhombicity sets in just below T HO , indicating that the lattice symmetry change is clearly associated with the hidden-order transition. Remarkably, unlike the continuous change expected in the order parameter at a second-order phase transition, δ ( T ) shows a sudden jump at T HO . This strongly suggests that the transition at T HO , which has been believed to be of second order, has a first-order nature. The fact that the latent heat has not been reported [1] , [2] , [3] , [14] indicates that the first-order nature is very weak; at T HO , the discontinuity of the order parameter that characterizes the low-temperature phase may be too small to be detected thermodynamically. These results lead us to conclude that the hidden-order transition is a weak first-order phase transition accompanied by lattice symmetry breaking from the fourfold tetragonal to twofold orthorhombic structure. The present result is consistent with the 29 Si NMR measurements under in-plane magnetic fields [8] , [18] , which reveal very similar temperature dependence of the spectral width having a clear jump at T HO ( Fig. 3d ). It has been suggested in a recent theory that the hyperfine fields at the Si site for an antiferroic multipole order that has an in-plane twofold anisotropy can lead to the NMR broadening below the transition [19] . Thus, this naturally implies a close correspondence between the orthorhombicity and NMR broadening as found in experiments. Two-dimensional diffraction profiles To verify that the peak split originates from the lattice symmetry change to the F mmm -type orthorhombic structure, we performed two-dimensional (2D) [ hk 0] scans near the (880) T Bragg peak ( Fig. 4 ). At 10 K below T HO , the data reveal a twin-peak structure ( Fig. 4a ) in contrast to the single peak above T HO ( Fig. 4b ). Here the integrated intensities above and below the transition are identical within experimental error, demonstrating that the twin peaks originate from the splitting of the (880) T Bragg peak. The elongated deformation along direction is due to worse resolution along this line as well as finite mosaicness inevitably present in the crystal. It should be stressed that the peak split along [ hh 0] direction found below T HO ( Fig. 4d ), which cannot be accounted for by the mosaicness, definitely indicates the appearance of two distinct lattice-plane spacings inside the crystal (reflecting the domain formation). We also find that along direction, although the peak does not show a clear split, it exhibits finite broadening below T HO ( Fig. 4e ). This indicates that the split occurs on two directions in the [ hk 0] plane, indicating that the single Bragg peak above T HO split into four peaks in the hidden-order phase. To show the consistency with the split into four peaks expected in the orthorhombic Fmmm -type structure [20] , [21] ( Fig. 1h ), we shift the high-temperature data at 19 K to four directions as sketched in the inset of Fig. 4c and add the four shifted data with the same weight. The calculated result shown in Fig. 4c is remarkably consistent with the measured data at 10 K ( Fig. 4a ). The line cuts of this result also reproduce the salient features of the 10-K data ( Fig. 4d,e ), namely the clear split along [ hh 0] and broadened peak along . The amount of the shifts in the calculation corresponds to the orthorhombicity δ =6.2 × 10 −5 , which is quantitatively consistent with the 2 θ / θ scan data in Fig. 3 . These results provide direct evidence that the lattice symmetry is lowered from the tetragonal I 4/ mmm to orthorhombic Fmmm -type with the formation of four domains, and that the fourfold rotational symmetry is broken at the hidden-order transition. 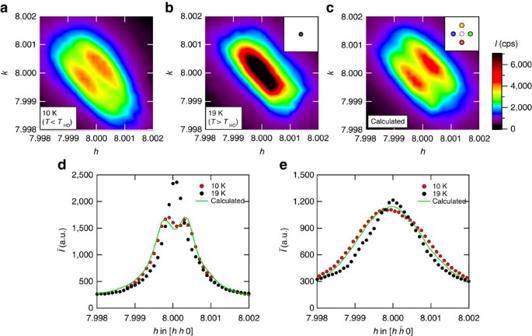Figure 4: 2D mapping of the (880)TBragg peak. (a) Data of [hk0] scan for 7.998≤h,k≤8.002 at 10 K belowTHO. (b) Data taken for the same range at 19 K aboveTHO. (c) Calculated results by using the 19-K data for the orthorhombicFmmmstructure with assumptions ofδ=6.2 × 10−5and equal volumes of four domains. The inset illustrates the assumed four positions (closed circles) shifted from the original tetragonal position (dashed circle), corresponding to the four domains in the orthorhombic phase (Fig. 1f). The colour bar indicates the intensity. (d) Line cuts along the [hh0] direction at 10 (red circles) and 19 K (blue circles), which are compared with the calculated one inc(green line). The intensityis averaged over a constant width ~0.0035 rlu along. (e) The same plot as indbut along the orthogonaldirection. Here the average is taken along [hh0]. Figure 4: 2D mapping of the (880) T Bragg peak. ( a ) Data of [ hk 0] scan for 7.998≤ h , k ≤8.002 at 10 K below T HO . ( b ) Data taken for the same range at 19 K above T HO . ( c ) Calculated results by using the 19-K data for the orthorhombic Fmmm structure with assumptions of δ =6.2 × 10 −5 and equal volumes of four domains. The inset illustrates the assumed four positions (closed circles) shifted from the original tetragonal position (dashed circle), corresponding to the four domains in the orthorhombic phase ( Fig. 1f ). The colour bar indicates the intensity. ( d ) Line cuts along the [ hh 0] direction at 10 (red circles) and 19 K (blue circles), which are compared with the calculated one in c (green line). The intensity is averaged over a constant width ~0.0035 rlu along . ( e ) The same plot as in d but along the orthogonal direction. Here the average is taken along [ hh 0]. Full size image The in-plane electronic anisotropy elongated along the [110] direction reported in the in-plane field rotation experiments [5] , [6] , [7] , [8] is fully compatible with this Fmmm -type space symmetry. It should be emphasized that the present results are obtained at zero field, demonstrating that such electronic nematicity is not field-induced. The formation of micro-domains evident from the multi-peak structure is also consistent with the above reports. We note that the intensity ratio of the two peaks is temperature-dependent ( Fig. 3a ), with the integrated intensity remaining unchanged ( Fig. 4a,b ). This suggests that the domain size and the position of domain walls change with temperature in the very clean crystal. This opens the possibility of ‘detwinning’ by an external force, which may be related to the recent report that the thermal expansion anomaly at T HO increases rapidly with application of extremely small in-plane uniaxial pressure [22] . The present results clarify the space symmetry of the hidden-order phase, which breaks fourfold rotational symmetry. This, along with the first-order nature revealed in this study, places very tight constraints on the genuine hidden-order parameter. Among the allowed irreducible representations for the hidden order (four non-degenerate A 1 , A 2 , B 1 and B 2 , and one degenerate E symmetries), the orthorhombic Fmmm -type space group symmetry pins down that the hidden order belongs to the E -type, more specifically E ( η a , η b ) with η a , η b =±1, in which the sign of η a η b determines the nematic direction of the domain [23] . Our results are consistent with the recently proposed orders that are compatible with this E -type symmetry [19] , [23] , [24] , [25] , [26] , [27] , [28] , [29] . Multipole orders with odd [19] , [24] , [28] (even [23] ) ranks with (without) time-reversal symmetry breaking should belong to E − ( E + ) symmetry, where the superscript sign represents the parity with respect to time reversal. More exotic orders, such as spin nematic [26] , [27] , hastatic [25] and dynamical circulating current orders [29] , are also consistent with the rotational symmetry breaking. The first-order nature of the hidden-order transition may also have an impact on the pressure phase diagram in URu 2 Si 2 . It has been discussed that the pressure-induced transition to the antiferromagnetic phase should be a first-order transition line, which ends when touching to the second-order hidden-order and antiferromagnetic transition lines at the bicritical point [4] . Now it is not required any more that the pressure-induced transition line should be the first-order. Experimental clarification on this point is a subject of future investigations. The magnitude of orthorhombicity δ is of the order of 10 −5 , which is two orders of magnitude smaller than that of similar structural transitions from the tetragonal I 4/ mmm to orthorhombic Fmmm phase in isomorphic BaFe 2 As 2 -based iron-pnictide superconductors [21] , [30] . This smallness of the lattice change implies that the hidden-order transition is driven by an electronic ordering, and small but finite electron-lattice coupling gives rise to the lattice distortion. It should be noted that in iron-pnictides the large orthorhombicity is believed to be associated with the ‘ferroic’ ( Q =0) orbital ordering, which is in sharp contrast to the URu 2 Si 2 case where the hidden order is most likely an antiferroic order with the wave vector Q =(001) [6] , [7] , [9] , [10] , [11] , [12] . Such an antiferroic ordering is expected to couple only weakly to the ferroic Q =0 orthorhombic distortion especially for high-rank multipole orders, in which the degree of local electronic distributions near the atoms are much smaller than that of dipoles in the antiferromagnetic case. We also note that in such a Q =(001) ordering, the staggered nature of the small local electronic distributions makes the two-colour crystallographic symmetry lower than the space symmetry, in which two-colour symmetry group should belong to a subgroup of Fmmm , such as Cmce -type (M.-T. Suzuki and H. Ikeda, personal communication). It has been reported that the temperature dependence of elastic constant ( C 11 − C 12 )/2 shows an anomalous softening [31] , [32] , but we point out that the elastic constants are also Q =0 quantities, which are hard to couple to the antiferroic high-rank mulitpole orders. This softening may be due to the incommensurate excitations found by neutron experiments [33] , which may also be related to the high-field incommensurate spin density wave phase identified above the critical field of hidden order [34] . In any case this anomaly does not appear to be closely related to the hidden order, because the ( C 11 − C 12 )/2 should be coupled to the orthorhombicity with Immm symmetry ( Fig. 1c,f,i ), which is not observed below T HO . Indeed it has been pointed out that the reported data of elastic constants may not be very useful for discrimination between the possible symmetries of hidden order [23] . Another remarkable finding is that the symmetry-breaking orthorhombic lattice distortion is quite sensitive to disorder ( Fig. 3a ). The fact that even the low-RRR samples exhibit clear signatures of the transition in the specific heat measurements [1] , [2] , [3] , [14] indicates that the gap formation itself by the Q =(001) band folding is a robust feature against disorder. In fact, this wave vector is determined by the nesting property of the Fermi surface [24] , [29] and hence should be insensitive to impurities. However, the transition temperature T HO shows a discernible decrease with lowering RRR particularly for samples with RRR ≲ 50 (ref. 14 ), which implies that impurities can perturb the hidden order. Further studies are required for a full understanding of the unusual impurity effect observed in the present study, but it may be related to the rotational degree of freedom of the nematic direction inside the ab plane in the degenerate E -type orders. The theoretical calculations for a rank-5 E − order without impurity scattering [24] have shown that the direction of the pseudospin is preferred to be along [110] than [100], but the energy difference between these two directions is very small. Then it is feasible that impurities can induce disorder in the nematic direction within the ab plane. Indeed, the recent analysis of the in-plane field-angle-dependent NMR results for the sample with RRR~70 by Kambe et al . [8] shows that there exists a noticeable distribution of the twofold anisotropic local fields, which leads to the Lorentzian line shape of the NMR spectra. Such impurity-induced disorder of the nematic direction may prevent the long-range lattice distortion through a nontrivial different- Q coupling between the antiferroic Q =(001) electronic order and the Q =0 orthorhombic distortion in the underlying lattice. Recent Landau free energy analysis indicates that a bilinear coupling of homogeneous stress to the staggered order parameter is forbidden by translational symmetry, and only higher order terms are present [35] . In such a case, a good coherency of the order (including the nematic direction) in a long range may be required to produce the observable lattice distortion. It may be helpful to note that an electronic nematic phase is also found in Sr 3 Ru 2 O 7 , where the nematic anisotropy is observed only in very clean samples [36] . In this case, the application of magnetic field is required to induce the nematic phase, and this field determines the nematic direction. When the impurity would disturb the nematic direction in such a condition, the order itself may be sensitive to disorder. Thus the impurity effects of nematic orders in strongly correlated electron systems appear to be an intriguing issue that deserves further investigations. Finally, our observation of the small but finite orthorhombic distortion in the clean crystal of URu 2 Si 2 pins down the space symmetry of the mysterious hidden order. For the full identification of the genuine order parameter, the next important issue is whether time reversal symmetry is broken or preserved in the hidden-order phase [18] , [37] , [38] . The observed unusual impurity effect implies that experiments using very clean samples would be quite important to clarify the nature of this enigmatic order. Sample preparation and characterisation High-quality single crystals of URu 2 Si 2 were grown by the Czochralski method in a tetra-arc furnace under argon gas atmosphere and subsequently purified by using the solid state electro-transport method under ultrahigh vacuum [14] . We used single crystals from two different batches, and the transport measurements in the crystals in these batches indicate that the residual resistivity ratios are RRR ~10 and ~670 respectively. The crystal structure analysis was performed by the synchrotron X-ray at SPring-8 (BL02B1). The sample was cut or crushed into small pieces and the crystalline quality of more than ~30 samples was checked at room temperature by using an imaging plate (IP). We have selected crystals with the sharpest Bragg spots at high angles for each batch. The selected best ultraclean crystal with RRR~670 used in this study has dimensions of ~70 × 50 × 30 μm 3 . Synchrotron X-ray measurements The temperature of the sample is controlled by a cryocooler equipped in the four-circle diffractometer. To expose a large portion of the crystal to the X-ray beam, we placed the sample on a fine silver wire (with a diameter of ~50 μm) attached to the cold head. The X-ray beam size is larger than the sample size. Typical Bragg peak profiles for (880) T the selected sample with RRR~670 at room temperature are shown in Fig. 2a and its inset, which are taken by the four-circle diffractometer at 17.15 keV and by the IP at 18.8 keV, respectively. We find no tails of the peak in any direction in the IP image, and similarly circular intensity profiles were obtained for four equivalent Bragg peaks (±8 ±8 0). In this IP resolution we are able to select samples with lattice constant distributions better than typical ones reported in the previous studies. To obtain a high resolution, we use a high-angle reflection set-up of four-circle diffractometer. The variable slits near the detector were set so that the angle resolution of Δ2 θ is as good as 0.008°. The resolution of lattice spacing Δ d / d can be strongly enhanced when 2 θ becomes close to 180°. We use a Si(311) monochrometer whose intrinsic energy resolution Δ E / E is ~ 2 × 10 −5 , which also contributes to the total experimental resolution. The calculated resolutions of lattice spacing Δ d / d as a function of angle for the IP and four-circle diffractometer are shown in Fig. 2b . Another important factor is the X-ray attenuation length. To see the splitting of the Bragg peak associated with the orthorhombic distortion, this length should be larger than the domain size. A comparison between the attenuation length and the expected 2 θ values for ( hh 0) T Bragg peaks ( Fig. 2c ) indicates that the choice of (880) T peak at X-ray energy of 17.15 keV satisfies both requirements of high resolution and long attenuation length. How to cite this article: Tonegawa, S. et al . Direct observation of lattice symmetry breaking at the hidden-order transition in URu 2 Si 2 . Nat. Commun. 5:4188 doi: 10.1038/ncomms5188 (2014).